Genome architecture is a selectable trait that can be maintained by antagonistic pleiotropy Chromosomal rearrangements are mutations contributing to both within and between species variation; however their contribution to fitness is yet to be measured. Here we show that chromosomal rearrangements are pervasive in natural isolates of Schizosaccharomyces pombe and contribute to reproductive isolation. To determine the fitness effects of chromosome structure, we constructed two inversions and eight translocations without changing the coding sequence. We show that chromosomal rearrangements contribute to both reproductive success in meiosis and growth rate in mitosis with a strong genotype by environment interaction. These changes are accompanied by alterations in gene expression. Strikingly, we find several examples leading to antagonistic pleiotropy. Even though chromosomal rearrangements may have a deleterious effect during sexual reproduction, some compensate with a strong growth advantage in mitosis. Our results constitute the first quantification of fitness effects caused by de novo mutations that result in chromosomal rearrangement variation and suggest a mechanism for their maintenance in natural populations. The first chromosomal rearrangement (CR) segregating in natural populations was described by Dobzhansky and Sturtevant [1] in Drosophila pseudoobscura . Genomes are now known to be far more fluid than was considered previously. CRs are widely distributed between species [2] , [3] and within species where they segregate as polymorphisms [4] , [5] . In humans, an increasing number of polymorphic variation for CRs is described in the literature [6] . One particular form of CRs, inversions, is often associated with adaptation to specific environments as observed in D . pseudoobscura [7] , Anopheles gambiae [8] and Mimulus guttatus [9] . The ubiquity of CRs and their consequent low hybrid viabilities [10] and reduced gene flow in heterozygotic crosses [7] , [11] has also led to the proposal that CRs serve as an initial genetic barrier in eukaryotic speciation [12] , [13] , [14] , [15] , [16] . In the well-documented cases of Drosophila and Anopheles , the frequency of CRs in the population varies clinally and/or seasonally, suggesting that the beneficial effects are caused by chromosome inversions. Several traits have since been associated with inversion polymorphisms [17] , [18] , indicating that they can influence the evolution of these populations. Yeast karyotypes have also been extensively characterized and similarly exhibit numerous CRs [19] . As an example, natural and industrial populations of Saccharomyces cerevisiae show remarkable chromosomal diversity [20] . In experimental evolution studies, the appearance of recurrent genomic rearrangements suggests that they increase fitness and are thus adaptive to laboratory conditions [21] , [22] . In most cases, growth advantages are caused by promoter modifications mediated either by reciprocal translocations that result in overexpression of metabolic genes [23] or duplication of genes important for specific growth conditions [24] . Thus, changes in fitness are often accompanied by changes in gene expression. In Drosophil a, different allozymes have been associated with particular chromosome inversions [25] , suggesting that gene expression differences are linked to these chromosomal configurations. Other examples of gene expression variation are caused by transposons [26] , gene duplications [27] and aneuploidies [28] . However, it is currently unknown whether the expression pattern is a direct consequence of structural variation per se or other nucleotide variation or a combination of both. Even though ample evidence exists for a direct role of CRs in adaptation, it is difficult to disentangle the contribution of gene alterations from their impact in chromosome structure as both often occur simultaneously. In this context, a key contribution by Colson et al. [29] demonstrated that two naturally occurring translocations may have been fixed between S. mikatae and S. cerevisiae by positive selection. The two reciprocal translocations of S. mikatae were ‘reconstructed’ in the S. cerevisiae genome in the absence of other polymorphisms and shown to provide growth advantages for S. cerevisiae in different environments. Thus, CRs can provide selective advantage in the absence of other forms of genome alterations. The results of Colson et al. [29] support a model where natural selection is responsible for the fixation of CRs between yeast species. However, the CRs tested in this study were naturally occurring and so we may expect them to be either neutral or advantageous, as strongly deleterious CRs are unlikely to be fixed in natural populations. Thus, the fundamental question remains to be answered: what are the fitness consequences of varying chromosome structure? Here we use the model organism S. pombe to investigate the phenotypic consequences of CRs that were engineered to mimic possible spontaneous mutations that only alter genome structure. Ten CRs, not previously tested by natural selection, were assayed for meiotic and mitotic fitness to unravel the contribution of CRs to population fitness variation across environments. We show that CRs display variation for both types of fitness measures and that they can be maintained in nature by a phenomenon called antagonistic pleiotropy. Natural chromosomal diversity impairs sexual reproduction S. pombe is an established model system for cellular and molecular biology due to its ease of genetic manipulation and conserved chromosomal organization. It has a small genome of ~14 Mbp distributed in three chromosomes of 5.7, 4.6 and 3.5 Mbp (ref. 30 ). As a result, S. pombe is a suitable organism to study the impact of chromosome structure in environmental adaptation and evolution. Given the importance and wide distribution of CRs in several species, we started by characterizing 10 natural isolates from different geographic regions ( Supplementary Table S1 ). L972 is the most widely used strain and the first to have its genome sequenced, thus we considered it as the reference genome. We analysed the karyotypic profile by whole-chromosome pulse-field gel electrophoresis (PFGE) and Not I restriction-PFGE followed by Southern blot analysis ( Fig. 1a–c ; Supplementary Figs S1–S3 ). Both whole chromosomes and Not I fragment sizes revealed a remarkable diversity for chromosome structure ( Fig. 1d ). In our small sample size, we have observed two independent translocations (NCYC132 and ATCC2476), a large inversion common to all except for L972 and other uncharacterised smaller intrachromosomal variations. 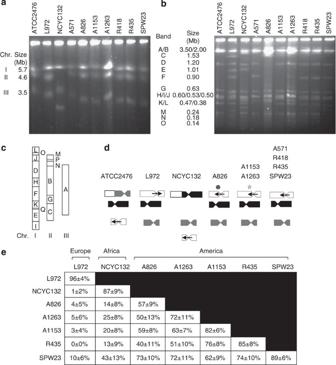Figure 1: Chromosomal analysis of natural isolates ofS. pombe. (a) Whole-chromosome PFGE analysis ofS. pombechromosomes. L972 reference strain contains three chromosomes: Chr. I 5.7 Mb, Chr. II 4.6 Mb and Chr. III 3.5 Mb. (b) PFGE of chromosomal DNA digested withNotI reveals different restriction patterns for each strain. The differences are not due toNotI polymorphisms, as all 13 are present and recognized byNotI enzyme (Supplementary Fig. S1). (c) Localization ofNotI restriction sites in reference strain L972. (d) Schematic representation of the three chromosomes in the different strains. Only the minimal CRs detected are represented (seeSupplementary Figs S2 and S3). These were mapped using chromosome-specific probes present at different positions, including the centromere-specific region imrL (imrL1, imrL2 and imrL3). Symbols in A1153, A1263 and A826 represent other not fully characterized CRs. (e) Meiotic viability of natural isolates. Each cross represents the analysis of 14–43 tetrads (containing the four meiotic products). Intervals correspond to 2 × s.e. for a binomial distribution. Figure 1: Chromosomal analysis of natural isolates of S. pombe. ( a ) Whole-chromosome PFGE analysis of S. pombe chromosomes. L972 reference strain contains three chromosomes: Chr. I 5.7 Mb, Chr. II 4.6 Mb and Chr. III 3.5 Mb. ( b ) PFGE of chromosomal DNA digested with Not I reveals different restriction patterns for each strain. The differences are not due to Not I polymorphisms, as all 13 are present and recognized by Not I enzyme ( Supplementary Fig. S1 ). ( c ) Localization of Not I restriction sites in reference strain L972. ( d ) Schematic representation of the three chromosomes in the different strains. Only the minimal CRs detected are represented (see Supplementary Figs S2 and S3 ). These were mapped using chromosome-specific probes present at different positions, including the centromere-specific region imrL (imrL1, imrL2 and imrL3). Symbols in A1153, A1263 and A826 represent other not fully characterized CRs. ( e ) Meiotic viability of natural isolates. Each cross represents the analysis of 14–43 tetrads (containing the four meiotic products). Intervals correspond to 2 × s.e. for a binomial distribution. Full size image We examined whether the observed chromosome variation was reflected at the sequence level. We measured a maximum local nucleotide diversity of 6.8 × 10 −3 ( Table 1 ) that is similar to the one found in a recent study using ca. 80 fission yeast natural isolates [31] . Both these and our results were corroborated by whole-genome quantification of nucleotide diversity performed in S. pombe [32] . Specifically, Rhind et al. [32] estimated 8.9 × 10 −3 nucleotide diversity from pairwise comparison of L972 and NCYC132 strains. This value is close to the one measured in worldwide populations of S. cerevisiae (5.6 × 10 −3 ) (ref. 33 ). Thus, not only do CRs appear to be pervasive in natural populations of S. pombe but, unpredictably, they keep nucleotide diversity levels close to those observed within-species ( Fig. 1 ; Table 1 ). Table 1 Nucleotide diversity for natural isolates. Full size table We next tested the genetic isolation between the natural isolates by scoring hybrid viabilities in pairwise crosses analysed by tetrad dissection. S. pombe is generally homothallic, implying that it is capable of switching between mating types and inbreeding. In order to directly measure genetic isolation, we required strains that stably express opposing mating types and so we disrupted the minimal sequence required for switching ( Supplementary Fig. S4 ) [34] . Expectedly, crosses within the same natural isolate showed high meiotic viability (>80%, Fig. 1e ). Different isolates from the same geographical location, which exhibit similar karyotypes, showed low levels of reproductive isolation ( Fig. 1e ; Supplementary Table S1 ). However, in spite of low genetic diversity, hybrid viability decreased sharply when we compared strains of different karyotypes (see L972 and NCYC132 as example; Fig. 1e ). These results point to CRs acting as genetic barriers, leading to low viability of hybrids. Consistently, CRs are considered early events for genetic isolation in chromosomal speciation models [16] . Artificial CRs affect meiotic viability It would be impossible to attribute the lower hybrid viability to CRs alone as all natural isolates possess further genetic differences. In addition, these CRs are a product of natural selection and therefore biased in their diversity. For this reason, we devised a set of newly generated yeast strains with unbiased CRs departing from a single genetic background. We produced two pericentric inversions and eight reciprocal translocations encompassing the three chromosomes using a Cre-loxP system developed by Molnar and Kleckner [35] ( Fig. 2a ; Supplementary Fig. S5 ). Our engineered strains are identical in their coding sequence, thus allowing us to investigate how chromosome structure affects fitness in an unbiased way. To control for non-specific Cre-loxP events, CRs were generated at least twice from each parental strain. We observed that all replicate CRs behaved identically, so we used them as replicates and averaged their results. 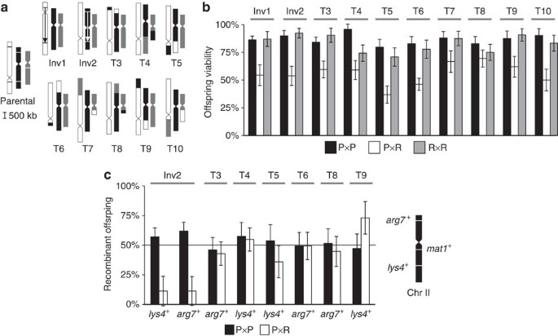Figure 2: Genetically engineered CRs reduce meiotic fitness. (a) Schematic representation of karyotypes for 10 different genetically engineeredS. pombestrains. All the strains are isogenic except for the rearrangement and its breakpoint. Chromosomes are drawn to scale. Inflexions represent the centromeres. To generate the CR strains, Cre recombinase was expressed in parental strains using a plasmid and selecting for two colonies, each representing a totally independent recombination event. (b) Meiotic viability of homozygotic and heterozygotic crosses. CRs reduce meiotic viability in heterozygotic crosses from 8 to 48% with the exception of T8 that exhibits no apparent reduction. Meiotic viability corresponds to the number of viable haploid spores that have formed a colony divided by the total number of spores. Each cross represents the analysis of 18–63 tetrads. Error bars represent 2 × s.e. for a binomial distribution. P—parental strain; R—rearranged strain. (c) Frequency of recombination between loci at the breakpoints and themat1locus. Inversions suppress recombination between any of the breakpoints and themat1locus by ~30%. In contrast, translocations do not significantly reduce recombination frequency. Only rearrangements involving chromosome II were scored. Error bars correspond to 2 × s.e. for a binomial distribution. Figure 2: Genetically engineered CRs reduce meiotic fitness. ( a ) Schematic representation of karyotypes for 10 different genetically engineered S. pombe strains. All the strains are isogenic except for the rearrangement and its breakpoint. Chromosomes are drawn to scale. Inflexions represent the centromeres. To generate the CR strains, Cre recombinase was expressed in parental strains using a plasmid and selecting for two colonies, each representing a totally independent recombination event. ( b ) Meiotic viability of homozygotic and heterozygotic crosses. CRs reduce meiotic viability in heterozygotic crosses from 8 to 48% with the exception of T8 that exhibits no apparent reduction. Meiotic viability corresponds to the number of viable haploid spores that have formed a colony divided by the total number of spores. Each cross represents the analysis of 18–63 tetrads. Error bars represent 2 × s.e. for a binomial distribution. P—parental strain; R—rearranged strain. ( c ) Frequency of recombination between loci at the breakpoints and the mat1 locus. Inversions suppress recombination between any of the breakpoints and the mat1 locus by ~30%. In contrast, translocations do not significantly reduce recombination frequency. Only rearrangements involving chromosome II were scored. Error bars correspond to 2 × s.e. for a binomial distribution. Full size image In order to test the meiotic fitness of artificial CRs, we performed pairwise crosses of parental with parental (P × P), parental with rearranged (P × R), and rearranged with rearranged (R × R) strains and quantified them by tetrad analysis. Offspring resulting from homozygotic crosses (P × P and R × R) were largely viable ( Fig. 2b ). The drop in viability for heterozygotic crosses (P × R) involving the two inversions was ~40%. Similarly, heterozygotic crosses involving translocations T3, T5, T6, T9 and T10 had losses in hybrid viability of 30–48%. Surprisingly, P × R crosses involving T8 did not lead to appreciable meiotic depression ( Fig. 2b ). As expected, meiotic recombination was unperturbed in homozygous crosses P × P but not in heterozygous crosses involving inversions ( Fig. 2c ). Overall, we observed genetic linkage of loci residing near the breakpoints of all the tested inversions and translocations ( Supplementary Fig. S6 ). Our results support previous observation for the reduction of gene flow inside pericentric inversions in Drosophila [36] . CRs are a selectable trait How can CRs be maintained as polymorphisms in nature if they impair meiosis? One possibility could be the occurrence of antagonistic pleiotropy during their life cycle, such that a given CR is disadvantageous in one part (meiosis) but then compensated by an advantageous trait in another (mitosis). To quantify mitotic fitness of the newly generated CRs, we performed competitive assays as described by Desai et al. [37] Briefly, the rearrangement and its parental ura4 + strain were competed against a control expressing GFP. The effect of the GFP was subsequently removed by subtracting the two selective coefficients (Δ S ): Details of the essay and calculations can be found in the Supplementary Information . We observed substantial variation for fitness associated with chromosome structure during the asexual life cycle in S. pombe ( Fig. 3a ). As an example, strains T6 and T9 exhibited growth advantage of 3% per generation when competed with the parental strain in rich medium (YES). In contrast, T5 and T8 showed growth disadvantage of 1.5% per generation. Strikingly, CRs can have very strong effects, either deleterious or beneficial even in a benign environment such as rich medium. 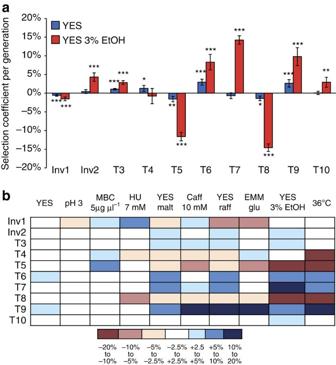Figure 3: Chromosome structure is a selectable trait. (a) Selective coefficients relative to the parentalura4+strain grown in rich media (YES) with and without 3% EtOH. Some CRs improve fitness relative to the parental, others are neutral or deleterious. Averages were calculated from >10 independent experiments each with two independent clones. These clones were generated by independent Cre-loxPrecombination events to minimize additional mutations and off-target effects. Error bars represent 2 × s.e. (***P<0.001, **P<0.01 and *P<0.05 according to Mann–WhitneyU-test). (b) Mitotic fitness in multiple environments of strains containing CRs. Modified strains display strong genotype by environment interactions. Selection coefficients are relative to parentalura4+strain. Coloured boxes represent average selection coefficient of designated CRs in each environment according to the scale represented at the bottom. Averages were calculated from >10 independent experiments each with two independent clones. Environments were ordered by increased variance in fitness. Figure 3: Chromosome structure is a selectable trait. ( a ) Selective coefficients relative to the parental ura4 + strain grown in rich media (YES) with and without 3% EtOH. Some CRs improve fitness relative to the parental, others are neutral or deleterious. Averages were calculated from >10 independent experiments each with two independent clones. These clones were generated by independent Cre- loxP recombination events to minimize additional mutations and off-target effects. Error bars represent 2 × s.e. (*** P <0.001, ** P <0.01 and * P <0.05 according to Mann–Whitney U -test). ( b ) Mitotic fitness in multiple environments of strains containing CRs. Modified strains display strong genotype by environment interactions. Selection coefficients are relative to parental ura4 + strain. Coloured boxes represent average selection coefficient of designated CRs in each environment according to the scale represented at the bottom. Averages were calculated from >10 independent experiments each with two independent clones. Environments were ordered by increased variance in fitness. Full size image As fitness effects are expected to change under different types of stress, we sought to assess fitness in several growth conditions. All of them, with the exception of YES, were suboptimal for the growth of a wild-type strain ( Supplementary Fig. S7 ). We additionally tested different carbon sources and other abiotic factors, such as low pH and increased temperature, mimicking environments that yeast may experience during fermentation. Our results show that, similar to other types of mutations, fitness effects conferred by CRs vary according to the environment in which they grow ( Fig. 3b ; Supplementary Fig. S8 ). The same rearrangement could be strongly beneficial in one environment but deleterious in another, exhibiting therefore genotype-by-environment interactions ( Fig. 3b ). Thus, our observations indicate that CRs not only affect growth but also they can be deleterious or beneficial depending on the environment that they are exposed. Antagonistic pleiotropy can maintain chromosomal diversity Next we tested directly whether advantageous CRs were always destined for fixation or whether their associated meiotic depression could keep them as polymorphism in the population via antagonistic pleiotropy. For this purpose, we devised an experiment where we mixed strains of both mating types either containing the CR or a GFP marker. We evolved these populations by serial passage under two growth conditions ( Fig. 4a ). Mixed populations were propagated either under an exclusively asexual life cycle (no mating), where the frequencies of the two genotypes would reflect their mitotic fitness differences, or a life cycle that included both asexual and sexual reproduction (with mating). We then tested for the maintenance of polymorphism of the CR under the two different environments, where it previously exhibited mitotic fitness advantage over its parental-GFP strain. We initiated these evolution tests introducing the CR at an initial frequency of ~25%, so that most crosses involving the CR strain were likely to be heterozygous. This way, we intended to mimic what may happen to an adaptive CR shortly after its appearance. As expected, in the absence of mating, the CR increased in frequency ( Fig. 4b ). If no other event takes place (such as de novo mutation), the CR would be expected to sweep through the population in a few hundred generations. However, when sexual reproduction occurs, the fixation of the CR was halted and its frequency was kept close to its initial levels ( Fig. 4b ; Supplementary Fig. S9 ). Thus, alternating the mode of reproduction prevented the extinction of the less-favoured genome configuration through antagonistic pleiotropy. 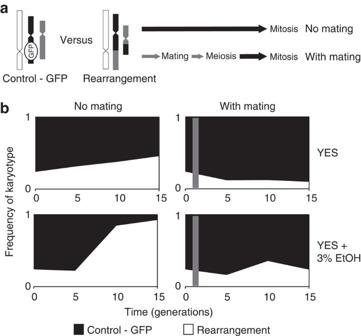Figure 4: Antagonistic pleiotropy can prevent selective sweeps of beneficial CRs. (a) Scheme of the evolution assay. The rearrangement T4 was mixed with its parentalura4+marked with GFP (Control-GFP) at a frequency of 25%. The mixture was evolved asexually for 3 days or 15 mitotic generations (no mating). In parallel, the same mixture was first grown in ME to induce random mating and meiosis (With mating). Meiotic products were germinated and further propagated for 15 generations of mitotic growth. Additional details can be found in theSupplementary Information. (b) Frequency of the rearrangement and Control-GFP strains in competition experiments. The graph represents the average of at least four replicates, which are displayed insupplementary Fig. S9. The top graphs show evolution in YES while the bottom graphs in YES+3% EtOH. Both environments are beneficial for the CR in relation to Control-GFP strain. Figure 4: Antagonistic pleiotropy can prevent selective sweeps of beneficial CRs. ( a ) Scheme of the evolution assay. The rearrangement T4 was mixed with its parental ura4 + marked with GFP (Control-GFP) at a frequency of 25%. The mixture was evolved asexually for 3 days or 15 mitotic generations (no mating). In parallel, the same mixture was first grown in ME to induce random mating and meiosis (With mating). Meiotic products were germinated and further propagated for 15 generations of mitotic growth. Additional details can be found in the Supplementary Information . ( b ) Frequency of the rearrangement and Control-GFP strains in competition experiments. The graph represents the average of at least four replicates, which are displayed in supplementary Fig. S9 . The top graphs show evolution in YES while the bottom graphs in YES+3% EtOH. Both environments are beneficial for the CR in relation to Control-GFP strain. Full size image One of the most important factors determining whether or not a CR is maintained in the population is the frequency of the rearrangement at the time of mating. A CR with a very large mitotic advantage is likely to reach frequencies of >50% and hence not pay any meiotic cost. In general, the maintenance of polymorphism or the fixation of one karyotype depends on the balance of the mitotic advantage, the meiotic depression and the frequency of CRs at the time of mating. We explored some of these effects in Supplementary Note 1 and Supplementary Fig. S10 . Given the effects of these variables, small demographic differences are likely to lead to very different outcomes in subpopulations exposed to the same environmental conditions, which may further contribute to the variability observed in natural S. pombe populations. CRs alter gene expression What was the basis of the growth differences in isogenic CR and parental strains? CRs confer structural changes to chromosomes that contribute to growth variability. In budding yeast, chromosome length is known to influence mitotic segregation and cell division [38] . Chromosomal size can also influence topological stress induced by DNA replication [39] . Thus, chromosome stability and, consequently, fitness is influenced by chromosome length. In order to test this hypothesis, we analysed strains containing the largest (6.96 Mb) and the smallest (1.93 Mb) chromosomes generated by this work (T7 and T8 respectively, Fig. 2a ; Table 2 ). If both topological stress and segregation stability were translated into slower growth, we would expect strains carrying longest chromosomes to have deleterious phenotypes even in rich media. However, T7 and T8 have overall opposite results for fitness in most tested conditions ( Fig. 3b ; Supplementary Fig. S8 ), arguing that chromosome size is not the major factor behind our observations. In addition, translocations where chromosome size is not significantly altered, such as T5, exhibit some of the most deleterious fitness effects ( Fig. 3b ; Supplementary Fig. S8 ). Table 2 Approximate chromosomal sizes of engineered chromosomal rearrangements. Full size table As all strains are isogenic, we hypothesized that fitness differences observed during asexual reproduction were caused by differences in gene expression near the breakpoints. The sites of recombination were introduced using an antibiotic resistance cassette ( Kan r ) that confers resistance to geneticin and can be used to assay for gene expression ( Fig. 5a ). Consistent with our hypothesis, we found that rearrangements respond differently to increasing amounts of geneticin ( Fig. 5b ). To directly evaluate differential gene expression near the breakpoints, we quantified mRNA levels of genes surrounding T5 and T7 ( Fig. 5c,d ). Out of four genes measured, expression of mrpl16 + was altered upon genome rearrangement ( Fig. 5d ). Together, our results indicate that CRs can lead to differences in gene expression near breakpoints. 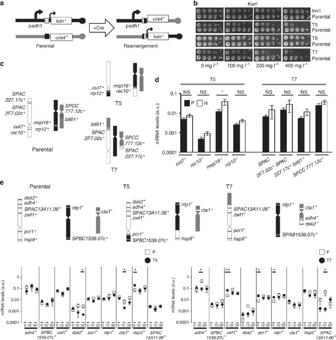Figure 5: Mitotic fitness of CRs varies in different environments. (a) Cre-loxP recombination scheme. Recombination between the promoter construct (padh1-loxP-kanMX6) and the gene construct (loxP-ura4-kanMX6) results in the formation of the rearrangement andura4+expression. Black and grey boxes represent loxP sequences and circles indicate centromeres. (b) T5 and T7 have lower expression of the antibiotic resistance geneKanrinserted near the breakpoint. Serial dilutions were spotted on plates containing 0, 100, 200 and 400 mg l−1ofgeneticinand allowed to grow for 4 days at 32 °C. (c) Schematic representation of genes near the breakpoints in the parental strain and their localization in T5 and T7. (d) CRs cause changes to expression of genes near breakpoints. mRNA levels relative to controls near the breakpoint. Gene expression was assayed in cells that have grown in rich media (YES). Error bars represent s.e. of three to six independent experiments. (*P<0.05 according to Mann–WhitneyU-test). (e) Schematic representation of genes involved in responses to general stress inS. pombe45and to ethanol stress inS. cerevisiae44in the parental strain and in T5 and T7. (f) Rearrangements cause changes in gene expression. T5 has lower gene expression upon exposure to 3% EtOH, whereas T7 is higher even before ethanol exposure. Genes are displayed by no particular order. Error bars represent s.e. of three to six independent experiments. Error bars represent s.e. (*P<0.05, **P<0.01 according to Mann–WhitneyU-test). In applying the very conservative Bonferoni correction, there is not enough power to detect statistical significance in our gene expression studies. Figure 5: Mitotic fitness of CRs varies in different environments. ( a ) Cre-loxP recombination scheme. Recombination between the promoter construct (padh1-loxP-kanMX6) and the gene construct (loxP-ura4-kanMX6) results in the formation of the rearrangement and ura4 + expression. Black and grey boxes represent loxP sequences and circles indicate centromeres. ( b ) T5 and T7 have lower expression of the antibiotic resistance gene Kan r inserted near the breakpoint. Serial dilutions were spotted on plates containing 0, 100, 200 and 400 mg l −1 of geneticin and allowed to grow for 4 days at 32 °C. ( c ) Schematic representation of genes near the breakpoints in the parental strain and their localization in T5 and T7. ( d ) CRs cause changes to expression of genes near breakpoints. mRNA levels relative to controls near the breakpoint. Gene expression was assayed in cells that have grown in rich media (YES). Error bars represent s.e. of three to six independent experiments. (* P <0.05 according to Mann–Whitney U -test). ( e ) Schematic representation of genes involved in responses to general stress in S. pombe [45] and to ethanol stress in S. cerevisiae [44] in the parental strain and in T5 and T7. ( f ) Rearrangements cause changes in gene expression. T5 has lower gene expression upon exposure to 3% EtOH, whereas T7 is higher even before ethanol exposure. Genes are displayed by no particular order. Error bars represent s.e. of three to six independent experiments. Error bars represent s.e. (* P <0.05, ** P <0.01 according to Mann–Whitney U -test). In applying the very conservative Bonferoni correction, there is not enough power to detect statistical significance in our gene expression studies. Full size image We then reasoned that fitness effects of individual CRs in response to multiple environments could be accompanied by differences in gene regulation beyond the breakpoints. There are several lines of evidence in the literature for the importance of chromosomal environment for gene expression [40] . For instance, studies comparing gene expression data from humans and chimpanzees highlight the importance of the alteration in genomic neighbourhoods as a factor that contributes to changes in gene expression levels [41] . Positional effects such as these can be translated into morphological and/or physiological variation with major implications for evolution [42] . Similarly, modifications in gene order and position by means of CRs should interfere with patterns of gene expression. To obtain direct evidence for this pattern, we selected two strains with opposing responses to 3% EtOH, a naturally occurring but restrictive environment for a fermenting organism such as fission yeast ( Fig. 3b ) [43] . Using qRT-PCR, we measured mRNA levels of the genes involved in stress and ethanol responses representative of different chromosomal locations [44] , [45] . Analysis of 21 genes revealed that not only gene expression was different between T5 and T7 exposed to 3% EtOH but, in some cases, these alterations preceded the environmental change ( Fig. 5e ; Supplementary Fig. S11 ). Strikingly, we found gene expression changes to occur in loci located several kilobases away from the breakpoint and even on different chromosomes ( Fig. 5e ). We were able to measure differences in gene expression in chromosomes that were not involved in the translocation, suggesting that CRs affect trans regulation and are therefore not restricted to the breakpoint area. Mating and meiosis are crucial evolutionary traits of yeasts in the wild. Not only they provide for new variants via chromosome assortment and recombination but also are tightly linked to the production of resistance spores under nutritional stress. As such, we expected that deviations to the predominant chromosome type would be lost shortly after their appearance. Surprisingly, we found extensive karyotype variability in natural populations of S. pombe . This led us to search for a mechanism that allows the maintenance of variation for chromosome structure. We produced new artificial CRs that do not disrupt the coding sequence and found significant differences in terms of their competitive fitness under mitotic growth. Despite encompassing large chromosome segments and thus affecting many genes, some CRs were beneficial, whereas others were neutral or deleterious. CRs that were beneficial during mitotic growth but had a meiotic cost constitute examples of antagonistic pleiotropy—whereby an allele (in this case a chromosome structure) is deleterious in one part of the life cycle (when mating at low initial frequency) and beneficial in another (asexual reproduction). In addition, the mitotic advantage of the rearrangements varies greatly with the environment, showing genotype-by-environment interactions. Thus, we propose that antagonistic pleiotropy provides a mechanism for karyotype diversity in natural populations. Although we understand well how the production of unbalanced chromosomes leads to the meiotic depression of rearrangements, mitotic advantages are more difficult to explain. We expect that changes in gene expression are likely to cause fitness variation among the different CR-containing strains. Thus, we favour a model whereby CRs disturb both cis and/or trans regulation, leading to variation in gene expression throughout the genome. It has been previously suggested that genomes are non-randomly arranged within the nuclear space forming chromosomal territories and giving rise to genomic neighbourhoods [40] . The nucleus has distinct structural and functional compartments and individual chromosomes can change their occupancy in the nucleus in order to accommodate specific expression profiles [40] . There is growing evidence that nuclear reorganization of chromosomes contributes to gene regulation caused by alterations in the relative position of genes to regulatory regions. One such example comes from studies in sensory neurons where the choice for expression of a particular odorant receptor results from the interaction of a single trans -acting enhancer element in chromosome 14 with the selected receptor in another chromosome [46] . Translocations and inversions change the localization and order of genes that can have profound effects on their expression. The three-dimensional (3D) configuration and chromosome dynamics are likely to change upon genome modifications. These alterations can cause modifications in gene expression by placing genes in a completely different constitutive heterochromatic or euchromatic region [47] or separating them from specific regulatory elements [48] . It is not currently known whether this type of long-range transcriptional regulation occurs in S. pombe. Such effects may even be negligible in fission yeast due to its small genome size and the fact that gene proximity is not always a requisite for coexpression [49] . Nonetheless, the CRs engineered by us are likely to modify the normal nuclear localization of genes (especially those closer to centromeres, telomeres and rDNA clusters) and possibly their heterochromatic state and, consequently, expression level. Another topic of current debate in the literature is the organization of genes into functional clusters likely maintained by natural selection [50] . Genome-wide expression studies in several organisms have shown that genes with similar expression patterns are arranged into clusters [51] , [52] . The expression of genes in these clusters is coordinated as the pattern of gene expression is similar for proximal genes [52] , [53] . Although the conservation of gene order appears to be the result of natural selection [50] , it is not clear that it is always associated with gene expression changes and related to functional constraints [54] . A recent study looking at gene expression in Drosophila male testis has shown that, at least for certain clusters of genes, disruption of gene organization does not lead to phenotypic alterations and that the cluster organization of genes is not necessary to achieve standard and coordinated gene expression levels [49] . One important difference in our work is that we have not disrupted any known gene cluster and, despite this, we observed substantial phenotypic diversity associated with small-scale gene expression differences. Overall, our results highlight the importance of genome architecture for fitness and establish a direct contribution of chromosome structure and gene organization. Using S. pombe as a model system, we show that variation in genome structure has fitness consequences as important as typical nucleotide changes. Our studies suggest that certain CRs may be maintained as polymorphisms in nature despite their low meiotic viability in heterozygotic crosses. Disadvantages in sexual cycle can be overcome by CR-dependent advantageous effects during asexual growth. Likewise, disadvantages in one environment can be balanced by advantages in another. These constitute unsuspected mechanisms of antagonistic pleiotropy capable of maintaining chromosome diversity in mixed populations. CRs can be fundamental for the generation of biological diversity at the karyotype level and may constitute a building block for further differentiation. Strains and media The strains used in this study are listed in Supplementary Tables S1, S2 . Standard media and growth conditions were used throughout this work [55] with minor modifications: arginine and lysine were added to all media and NH 4 + was used at a final concentration of 225 mg l −1 in all EMM-based media. Cultures were grown in rich media (YES) or minimal media (EMM) at 32 °C with shaking, unless otherwise stated. Tetrad dissection for meiotic viability analysis was performed on YES solid media. Construction of a non-exchangeable mating type cassette In order to fix the mating type in natural isolates, a stable non-switchable mat1 locus was constructed both for mat1-P and mat1-M as described previously [34] . Briefly, the pFA6a-natMX6 plasmid was used as backbone for the insertion of fragments PCR1 and PCR2 ( Supplementary Fig. S4 ). Sequences of mat1-M , mat1-P , H2 and H1 were taken from Kelly et al. [56] PCR1 and PCR2 products were amplified from pON104 ( mat1-P ) and pON107 ( mat1-M ) plasmids, kindly provided by Olaf Neilsen (University of Copenhagen). The final constructs, pcr1P-natMX6-pcr2P and pcr1M-natMX6-pcr2M, were used to transform homothallic S. pombe . To confirm loss of the switching capacity, strains were plated in maltose extract agar (ME) for 3 days and checked for the absence of mating and meiotic products. Meiotic viability Meiotic crosses were executed as described in Moreno et al. [55] Tetrad dissections were performed on YES plates in a micromanipulator equipped with a glass needle (Singer Instruments). Meiotic viability is given as the number of colonies formed by each meiotic product divided by the total number of colonies expected. Pulse-field gel electrophoresis PFGE was performed as described by Ferreira and Cooper [57] using exponentially growing cells (0.5–1 × 10 7 cells per ml) in YES media. All PFGE were performed on a Biorad CHEF-DR III System. DNA was visualized by ethidium bromide staining and gels were processed for Southern blotting. Southern blot analysis Southern blot analysis was performed as described by Ferreira and Cooper [57] . Different probes were labelled with 32 P-dCTP using the Prime-it II random primer labelling kit (Stratagene). Probes were generated by PCR amplification ( Supplementary Table S3 ). DNA sequencing and alignment Colony PCR was performed to obtain genomic DNA for PCR amplification ( Supplementary Table S3 ). Genetic sequences were amplified with Roche PCR master mix (Roche) and purified with Promega Wizard SV Gel and PCR clean up system. DNA sequencing was performed according to the manufacter’s instructions using the BigDye Terminator v1.1 Cycle Sequencing Kit (Applied Biosystems). Analysis of DNA sequences and their quality were performed using 4Peaks and DNAStrider software, respectively. DNA sequence alignment was performed in MUSCLE from EBI and π values calculated using DnaSP [58] . Construction of CR strains For parental strains, different combinations of Molnar and Kleckner’s [35] strains were crossed to obtained different haploid strains with selected combination of the loxP cassette at the auxotrophic marker ( Supplementary Fig. S2 ; Supplementary Table S2 ). MGF1070 and MGF2098 were generated by protoplast fusion of strains MGF539 and MGF542 as described by Gingold [59] . For sporulation of the diploids, cells were transformed with the pON104 plasmid. With the exception of MGF1070 and MGF2098, all strains were transformed independently with mat1-M and mat1-P fragments to fix their mating types. Strains were selected based on the simultaneous presence of padh1-loxP-kanMX6 and loxP-ura4-kanMX6 fragment after PCR amplification. These strains are referred to as parental strains. For generation of rearranged strains, parental strains were transformed with pREP81-Cre or pREP81 plasmids and plated directly in selective media EMM–leu with 4 mM thiamine. Single colonies were inoculated overnight in liquid media EMM–leu and plated in EMM–ura 18/20 h after for selection of the recombination event. Single colonies were then re-streaked into EMM–ura and then to YES and genotyped. We selected two colonies, each representing a totally independent recombination event. All the strains were frozen immediately as soon as the genotype was confirmed. Cells were exposed to the minimum possible time to the Cre recombinase, by promoting the loss of the pREP81–Cre plasmid straight after the recombination event. As parental strains are ura4 − and CRs are ura4 + , we obtained equivalent strains ura4 + (termed Parental ura4 + strains) to use in competition assays. To generate these strains, the same parental cells that were used for pREP81-Cre transformation were crossed with strain L972 or another prototrophic strain. GFP tagged cells were created by insertion of 3nmt1-GFP-hphMX6 fragment [60] near the breakpoint loci ( Supplementary Table S1 ). Competitive fitness assays To measure the fitness effects of CRs, we developed a FACS-based competitive assay. Unlabelled CR strain and Parental ura4 + strain were independently competed against its reference GFP-labelled strain (Control-GFP, Supplementary Fig. S2 ). To do so, both CR and control strain were grown in YES liquid medium for 24 h at 32 °C with aeration and shaking. The following day cultures were diluted and, once in mid-exponential phase, mixed at 1:1 ratios with the fluorescently labelled control strain with total initial cell density in the order of 2 × 10 5 cells per ml. The effective ratio of the mixture was measured using FACS. Then, 600 μl of the mix was placed in a 96-deep-well plate and incubated in a mini-shaker (VWR) at 32 °C with 850 r.p.m. agitation. Unless otherwise stated, cells were grown at 32 °C. Every 24 h cells were diluted 1:30 to fresh media. This was repeated three times. After 4 days (~20 generations), final ratios of unlabelled to GFP-labelled strain were measured. The number of GFP-positive (reference) and non-fluorescent (experimental) cells was determined using a Cyan ADP Cell Analyzer (Beckman Coulter, Inc.) counting 10,000 total cells for each sample. Selection coefficients (Δ S ) were calculated as: with t 0 the initial time (zero generations) and t f the final time (20 generations). In order to obtain the selection coefficient of the rearrangement, we extracted the weight of the GFP, such that the final selection coefficient is given by: The selection coefficient was estimated as an average of at least 20 independent competition assays. Assaying for antagonistic pleiotropy T4, T10 and their respective controls were transformed as described above to create the set of four strains used in the experiment: h − CR, h + CR, h − Control-GFP and h + Control-GFP. These strains were grown separately two overnights in either YES or YES+3% EtOH. Then, h − CR and h + CR were mixed in equal proportions, and the same was done for the control-GFP strains. Finally, the CR mix and control-GFP mix were mixed such that the CR was at a low frequency (~20%). The frequencies were measured by flow cytometry using an LSR Fortessa (BD Biosciences), producing point 0 in Fig. 4 and Supplementary Fig. S6 . Here the mixtures were split in two different plates. A 96-deep-well plate with either YES or YES+3% EtOH and a ME 96-well plate. The first plate corresponds to the CR dynamics without mating and was incubated at 32 °C during 24 h, at which point the cells were diluted into fresh medium and their frequency measured. This was done over 3 days. The second plate corresponds to the mating scenario and was incubated at 25 °C for 3 days, when tetrad production was checked. Spores and cells were harvested and incubated in water with 1% Hellix pomatia extract at room temperature for 16 h to digest all vegetative cells and release the spores. The spores were washed in water and resuspended in YES, incubated overnight at 32 °C and then diluted (20–600 μl) in either YES or YES+3% EtOH. This was repeated for 3 days. qRT-PCR analysis of gene expression Total RNA was isolated from exponentially growing cultures of each strain using a RiboPure-Yeast kit (Ambion). Gene expression was assayed in cells that have grown in YES and after 15- or 30-min exposure to 3% EtOH. Synthesis of cDNA was performed using MMLV Reverse Transcriptase (Promega). Quantitative PCR was performed using SYBR Green PCR Master Mix (Applied Biosystems) following the manufacturer’s instructions. All qPCR reactions were performed in a final volume of 10 μl, three replicates per sample (technical replicas), and set up in a 384-well plate. Quantitative DNA amplification was carried out in the ABI 7900 HT machine (Applied Biosystems). Reporter signals were analysed using SDS 2.4 software (Applied Biosystems). The C T value of the gene coding for actin ( act1 + ) was used for the normalization of variable cDNA levels and induction factors were determined for each gene and condition. Growth assays Strains were grown overnight in YES in a volume of 600 μl per well in 96-deep-well plates. The following day, cells were diluted 1:30 to the appropriate media and time points were recorded approximately every 2 h. Cell OD was measured in a final volume of 100 μl in 96-well flat bottom at 600 nm in Victor III apparatus (Perkin Elmer). Viability assays Drug sensitivity analysis was performed as described [55] . Briefly, exponentially growing cells in YES media were collected and counted. Five-fold serial dilutions from a starting concentration of 1 × 10 7 cells per ml are prepared and 5-μl spots of the serial dilutions are spotted into the specific media containing agar plate. How to cite this article: Avelar, A. T. et al. Genome architecture is a selectable trait that can be maintained by antagonistic pleiotropy. Nat. Commun. 4:2235 doi: 10.1038/ncomms3235 (2013).